Mean-field theory of random close packings of axisymmetric particles Finding the optimal random packing of non-spherical particles is an open problem with great significance in a broad range of scientific and engineering fields. So far, this search has been performed only empirically on a case-by-case basis, in particular, for shapes like dimers, spherocylinders and ellipsoids of revolution. Here we present a mean-field formalism to estimate the packing density of axisymmetric non-spherical particles. We derive an analytic continuation from the sphere that provides a phase diagram predicting that, for the same coordination number, the density of monodisperse random packings follows the sequence of increasing packing fractions: spheres <oblate ellipsoids <prolate ellipsoids <dimers <spherocylinders. We find the maximal packing densities of 73.1% for spherocylinders and 70.7% for dimers, in good agreement with the largest densities found in simulations. Moreover, we find a packing density of 73.6% for lens-shaped particles, representing the densest random packing of the axisymmetric objects studied so far. Understanding the properties of assemblies of particles from the anisotropy of their building blocks is a central challenge in materials science [1] , [2] , [3] . In particular, the shape that leads to the densest random packing has been systematically sought empirically [4] , [5] , [6] , [7] , [8] , [9] , [10] , [11] , [12] , [13] , [14] , [15] , [16] , [17] , as it is expected to constitute a superior glass forming material [1] . Despite the significance of random packings of anisotropic particles in a range of fields like self-assembly of nanoparticles, liquid crystals, glasses and granular processing [18] , there is yet no theoretical framework to estimate their packing density. Thus, random packings of anisotropic particles are typically investigated on a case-by-case basis using computer simulations, which have shown, for example, that elongated shapes like prolate ellipsoids and spherocylinders can pack considerably denser than the random close packing (RCP) fraction of spheres at RCP ≈0.64. These shapes exhibit a maximum in the packing fraction for aspect ratios (length/width) close to the sphere [4] , [5] , [6] . 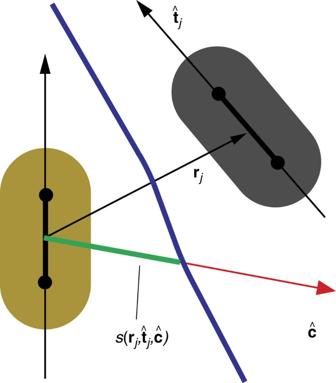Figure 1: Parametrization of the VB. The VB in blue, denoted by, along a directionbetween two spherocylinders of relative positionrjand orientation. Table 1 summarizes the empirical findings for maximal densities and highlights a further caveat of simulation and experimental studies: The protocol dependence of the final close-packed (or jammed) state leading to a large variance of the maximal packing fractions found for the same shape. This observation can be explained using the picture of a rugged energy landscape from theories of the glass phase [19] . Different algorithms get stuck in different metastable basins of the energy landscape, reaching different final packing states. Table 1 Overview of packing fractions from simulations and experiments. Full size table Here we present a mean-field approach to systematically study the packing fraction of a class of anisotropic shapes with rotational symmetry, which can therefore guide further empirical studies. Explicit results are obtained for axisymmetric particles like dimers, spherocylinders and lens-shaped particles, and we discuss generalizations to other shapes like tetrahedra, cubes and irregular polyhedra. Furthermore, we derive an analytic continuation of the spherical RCP which provides a phase diagram for these and other anisotropic particles like oblate and prolate ellipsoids. We first define the Voronoi volume of a non-spherical particle on which our calculation is based, and show that it can be calculated analytically for many different shapes by a decomposition of the shape into overlapping and intersecting spheres, which we organize into interactions between points, lines and anti-points. We then develop a statistical mean-field theory of the Voronoi volume to treat the particle correlations in the packing. This geometric mean-field approach is complemented by a quantitative estimation of the variation of the average contact number with the particle aspect ratio. The predicted packing density is interpreted as an upper bound of the empirically obtained packings. Voronoi boundary between non-spherical objects We consider rotationally symmetric objects for which the aspect ratio α is defined as length/width, where the length is measured along the symmetry axis. In the following, we focus on the region 0<α<2, where the largest densities are found [17] . Our description of packings relies on a suitable tessellation of space into non-overlapping volumes [20] . We use the standard Voronoi convention [21] , [22] , where one associates with each particle the fraction of space that is closer to this particle than to any other one. This defines the Voronoi volume W i of a particle i , which depends on the configurations of all particles (including position r and orientation ). The total volume V occupied by N particles is , and the packing fraction of monodisperse particles of volume V α and aspect ratio α follows as = NV α / V . In order to determine W i one has to know the Voronoi boundary (VB) between two particles i and j , which is the hypersurface that contains all points equidistant to both particles ( Fig. 1 for spherocylinders). The VB of the volume W i along , denoted by , is the minimal one in this direction among all possible VBs of each particle j in the packing. It is formally obtained by the global minimization [20] : Figure 1: Parametrization of the VB. The VB in blue, denoted by , along a direction between two spherocylinders of relative position r j and orientation . Full size image where denotes the VB along between particles i and j with relative position r j and orientation ( Fig. 1 ). The Voronoi volume follows then exactly as the orientational integral, The VB between two equal spheres is identical to the VB between two points and is a flat plane perpendicular to the separation vector ( Fig. 2a ) [20] . Finding the VB for more complicated shapes is a challenging problem in computational geometry, which is typically only solved numerically [23] . We approach this problem analytically by considering a decomposition of the non-spherical shape into overlapping spheres. The VB is then determined as follows: Every segment of the VB arises due to the Voronoi interaction between a particular sphere on each of the two particles reducing the problem to identifying the correct spheres that interact. This identification follows an exact algorithm for a large class of shapes obtained by the union and intersection of spheres, which can be translated into an analytical expression of the VB as outlined in Fig. 3 for dimers, spherocylinders and lens-shaped particles. 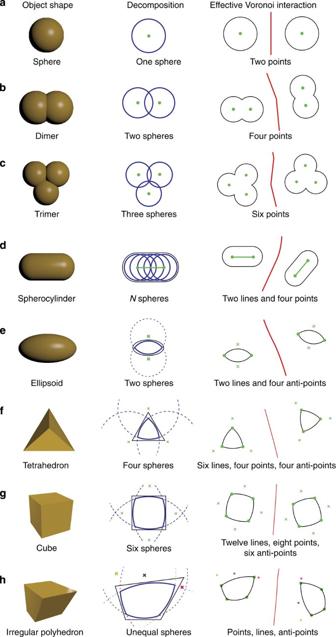Figure 2: Decomposition of various shapes and effective Voronoi interactions. Arbitrary object shapes can be decomposed into unions and intersections of spheres. (a–d) Union of spheres. The VB between two such objects is equivalent to the VB between the point multiplets at the centre of the spheres, as shown for four basic shapes. (e–g) Intersection of spheres. The VB between such intersections is equivalent to that between multiplets of ‘anti-points’ at the centre of the spheres, indicated by crosses, and, in addition, lines at the edges of the intersections, shown as points ine–d. The additional lines arise due to the positive curvature at the singular intersections, resulting in edges that point outwards from the particle rather than inwards. In the case of dimers and trimers shown inb,c, the curvature is negative and the edges do not influence the VB. The generalization to (f) tetrahedra-like, (g) cubes and (h) irregular polyhedra-like shapes is straightforward. Note that the VBs drawn ine–hare only qualitative. Figure 2: Decomposition of various shapes and effective Voronoi interactions. Arbitrary object shapes can be decomposed into unions and intersections of spheres. ( a – d ) Union of spheres. The VB between two such objects is equivalent to the VB between the point multiplets at the centre of the spheres, as shown for four basic shapes. ( e – g ) Intersection of spheres. The VB between such intersections is equivalent to that between multiplets of ‘anti-points’ at the centre of the spheres, indicated by crosses, and, in addition, lines at the edges of the intersections, shown as points in e – d . The additional lines arise due to the positive curvature at the singular intersections, resulting in edges that point outwards from the particle rather than inwards. In the case of dimers and trimers shown in b , c , the curvature is negative and the edges do not influence the VB. The generalization to ( f ) tetrahedra-like, ( g ) cubes and ( h ) irregular polyhedra-like shapes is straightforward. Note that the VBs drawn in e – h are only qualitative. 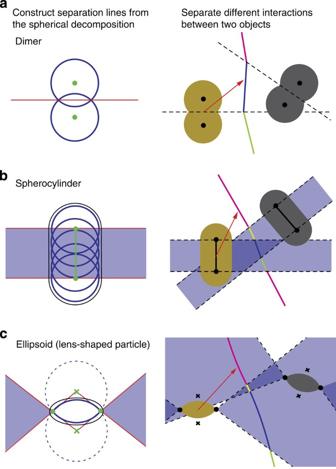Figure 3: Analytical solution to determine the VB for non-spherical objects. (a) The VB between the two objects of a given relative position and orientation consists of the VBs between particular spheres on each of the two objects. The spheres that interact are determined by separation lines given as the VBs between the spheres in the filling. For dimers, there is one separation line for each object, tesselating space into four areas, in which only one interaction is correct. The pink part ina, for example, is the VB between the two upper spheres. (b) The dense overlap of spheres in spherocylinders leads to a line as effective Voronoi interaction at the centre of the cylindrical part. This line interaction has to be separated from the point interactions due to the centres of the spherical caps as indicated. Overall, the two separation lines for each object lead to a tessellation of space into nine different areas, where only one of the possible line–line, line–point, point–line, and point–point interactions is possible. The yellow part inb, for example, is due to the upper point on spherocylinder 1 and the line of 2. Regions of line interactions are indicated by blue shades. (c) The spherical decomposition of ellipsoid-like shapes is analogous to dimers, only that now the opposite sphere centres interact. We indicate this inverted interaction by a cross at the centres of the spheres and refer to these points as ‘anti-points’. In addition, the positive curvature at the intersection point leads to an additional line interaction, which is a circle in 3D (a point in 2D) and indicated here by two points. The separation lines are then given by radial vectors through the intersection point/line. The Voronoi interaction between the two ellipsoids is thus given by two pairs of two anti-points and a line, which is the same class of interactions as spherocylinders. The different point and line interactions are separated analogous to spherocylinders, as shown. Full size image Figure 3: Analytical solution to determine the VB for non-spherical objects. ( a ) The VB between the two objects of a given relative position and orientation consists of the VBs between particular spheres on each of the two objects. The spheres that interact are determined by separation lines given as the VBs between the spheres in the filling. For dimers, there is one separation line for each object, tesselating space into four areas, in which only one interaction is correct. The pink part in a , for example, is the VB between the two upper spheres. ( b ) The dense overlap of spheres in spherocylinders leads to a line as effective Voronoi interaction at the centre of the cylindrical part. This line interaction has to be separated from the point interactions due to the centres of the spherical caps as indicated. Overall, the two separation lines for each object lead to a tessellation of space into nine different areas, where only one of the possible line–line, line–point, point–line, and point–point interactions is possible. The yellow part in b , for example, is due to the upper point on spherocylinder 1 and the line of 2. Regions of line interactions are indicated by blue shades. ( c ) The spherical decomposition of ellipsoid-like shapes is analogous to dimers, only that now the opposite sphere centres interact. We indicate this inverted interaction by a cross at the centres of the spheres and refer to these points as ‘anti-points’. In addition, the positive curvature at the intersection point leads to an additional line interaction, which is a circle in 3D (a point in 2D) and indicated here by two points. The separation lines are then given by radial vectors through the intersection point/line. The Voronoi interaction between the two ellipsoids is thus given by two pairs of two anti-points and a line, which is the same class of interactions as spherocylinders. The different point and line interactions are separated analogous to spherocylinders, as shown. Full size image For instance, a dimer is the union of a pair of spheres ( Fig. 2b ). The dimers VB is thus a composition of maximal four different surfaces depending on the relative orientation of the dimers defined by four points at the centre of each sphere ( Fig. 3a ). The extension to trimers is straightforward ( Fig. 2c ). Likewise, n overlapping spheres lead to compositions of n surfaces. A spherocylinder is a dense overlap of spheres of equal radii and the VB interaction is identical to that between four points and two lines ( Fig. 2d ). The interactions then simplify into line–line, line–point, and point–point interactions, which generally lead to a curved VB for non-parallel orientations ( Fig. 3b ). The Voronoi decomposition used for dimers and spherocylinders can be generalized to arbitrary shapes by using a dense filling of spheres with unequal radii [24] . However, even if it is still algorithmically well defined, this procedure may become practically tedious for dense unions of polydisperse spheres. Alternatively one can apply specialized algorithms to compute numerical VBs between curved line segments [25] . Here we propose an analytically tractable approach: Convex shapes can be approximated by intersections of a finite number of spheres. An oblate ellipsoid, for example, is well approximated by a lens-shaped particle, which consists of the intersection of two spheres; an intersection of four spheres is close to a tetrahedra, and six spheres can approximate a cube. This is illustrated in Fig. 2e–h , and the corresponding algorithms outlined in Fig. 3c . The main insight is that the effective Voronoi interaction of these shapes is governed by a symmetry: Points map to ‘anti-points’ (as the interactions between spheres is inverted; Fig. 3c ). The VB of ellipsoid-like objects arises from the interaction between four anti-points and four points in two dimensions ( Fig. 3c ) or lines in three dimensions, and thus falls into the same class as spherocylinders. For cubes, the effective interaction is that of twelve lines, eight points and six anti-points ( Fig. 2g ). Analytic expressions of the VB for dimers and spherocylinders are calculated in the Supplementary Methods . A statistical theory for Voronoi volume fluctuations We turn the above formalism into a mean-field theory to calculate the volume fraction of a packing of monodisperse non-spherical objects. In order to take into account multi-particle correlations in the packing, we use a statistical mechanics treatment where the overall volume is expressed in terms of the average Voronoi volume : (ref. 20 ) characterized by the average coordination number z , which denotes the mean number of contacting neighbours in the packing. This approach is motivated by the observation that, as N →∞, packings exhibit reproducible phase behaviour, which is characterized by only few observables such as and z (ref. 26 ). Our statistical mechanics framework is based on the Edwards ensemble approach, which considers the volume as a Hamiltonian of the system and attempts to find the minimum volume [27] . Here is given as the ensemble average of W i over all particles in the packing: . We obtain therefore from equation (2): In the last step, we have introduced the probability density p ( c ), which contains the probability to find the VB at c in the direction . The lower integration limit is the minimal value of the boundary along , which corresponds to the hard-core boundary of the particle in that direction. We introduce the cumulative distribution function (CDF) P ( c ) via the usual definition . Substituting the CDF in equation (3) and performing an integration by parts leads to the volume integral where we indicate the dependence on z . In a geometric picture [20] , P ( c , z ) is interpreted as the probability that N −1 particles are outside a volume Ω centred at c (see Fig. 4 ), as otherwise they would contribute a shorter VB. 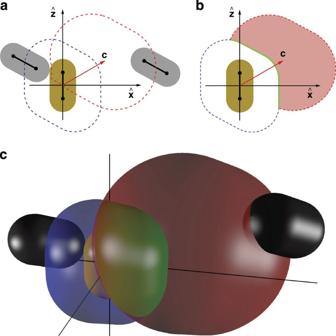Figure 4: The Voronoi excluded volume and surface. (a) The hard-core repulsion between the two objects defines the hard-core excluded volumeVex(enclosed by a dashed blue line): This volume is excluded for the centre of mass of any other object. Packings of rods in the limitα→∞ can be described by a simple random contact equation based onVex(ref.51). We introduce the Voronoi excluded volume Ω (enclosed by a dashed red line), which is the basis of our statistical theory of the Voronoi volume. The volume Ω, equation (5), is excluded by the condition that no other particle should contribute a VB smaller thancin the direction, which defines the CDFP(c,z). (b) Taking into account the hard-core exclusion leads to the effective Voronoi excluded volumeV* (indicated as red volume), which is excluded for bulk particles. Likewise, the overlap ofVexand Ω excludes the surfaceS* (thick green line) for all contacting particles. The volumes are shown here for a single orientation. (c) The 3D plot corresponding tob: The central particle is in brown,Vexis indicated in blue,V* in red, andS* in green. This leads to the definition Figure 4: The Voronoi excluded volume and surface. ( a ) The hard-core repulsion between the two objects defines the hard-core excluded volume V ex (enclosed by a dashed blue line): This volume is excluded for the centre of mass of any other object. Packings of rods in the limit α →∞ can be described by a simple random contact equation based on V ex (ref. 51 ). We introduce the Voronoi excluded volume Ω (enclosed by a dashed red line), which is the basis of our statistical theory of the Voronoi volume. The volume Ω, equation (5), is excluded by the condition that no other particle should contribute a VB smaller than c in the direction , which defines the CDF P ( c , z ). ( b ) Taking into account the hard-core exclusion leads to the effective Voronoi excluded volume V * (indicated as red volume), which is excluded for bulk particles. Likewise, the overlap of V ex and Ω excludes the surface S * (thick green line) for all contacting particles. The volumes are shown here for a single orientation . ( c ) The 3D plot corresponding to b : The central particle is in brown, V ex is indicated in blue, V * in red, and S * in green. Full size image where Θ( x ) denotes the usual Heavyside step. We refer to Ω as the Voronoi excluded volume, which extends the standard concept of the hard-core excluded volume V ex considered by Onsager in his theory of elongated equilibrium rods [28] ( Fig. 4 ). The dependence of P ( c , z ) on Ω has been treated at a mean-field level in Song et al . [20] and has been derived from a theory of correlations using liquid state theory in [29] for high-dimensional sphere packings. In both cases it provides a Boltzmann-like exponential form in the limit N →∞, where ρ ( r , z ) is the density of spheres at r . The crucial step is to generalize this result to anisotropic particles. Following Onsager [28] , we treat particles of different orientations as belonging to different species. This is the key assumption to treat orientational correlations within a mean-field approach. Thus, the problem for non-spherical particles can be mapped to that of polydisperse spheres for which P factorizes into the contributions of the different radii [30] . We thus obtain the factorized form: where is the density of particles with orientation at r . Next, we assume an approximation of this density in terms of contact and bulk contributions, which is motivated by the connection with the radial distribution function in spherical theories in both high and low dimensions [20] , [29] . The contact contribution relies on the condition of contact between the two particles of a given relative position r and orientation , which defines the contact radius : is the value of r for which the two particles are in contact without overlap. In the case of equal spheres the contact radius is simply . For non-spherical objects, depends on the object shape and the relative orientation ( Supplementary Methods ). Using we can separate bulk and contact terms in as in [20] , [29] : The prefactor 1/4π is the density of orientations, which we assume isotropic. The symbols and σ ( z ) stand for the average free-volume of particles in the bulk and the average free-surface of particles at contact, respectively, which are discussed further below. The approximation equation (7) corresponds to considering a pair distribution function as a delta function modelling the contact particles plus a constant term modelling the particles in the bulk [29] , which are thus considered as a uniform structure. These assumptions are further tested in the Methods section. Substituting equation (7) into equation (6) leads to our final result for the CDF: Here we have explicitly written the dependence of on , which is important to interpret equation (4) as a self-consistent equation to obtain the volume fraction of the packing. The free-volume per particle in the bulk depends specifically on as The CDF thus factorizes into two contributions: A contact term: and a bulk term: such that The volume V * is the volume excluded by Ω for bulk particles and takes into account the overlap between Ω and the hard-core excluded volume V ex : , where denotes an orientational average. Likewise, S * is the surface excluded by Ω for contacting particles: , where ∂V ex denotes the boundary of V ex . The volumes V ex and Ω as well as the resulting V * and S * are calculated in the Supplementary Methods and shown in Fig. 4 for spherocylinders. The surface density σ( z ) is a measure for the available surface for contacts when the packing is characterized by an average coordination number z . We evaluate this density by simulating random local configurations of one particle with z non-overlapping contacting particles and determining the average available free-surface. This surface is given by S *( c m ), where c m is the minimal contributed VB among the z contacts in the direction . Averaging over many realizations with a uniform distribution of orientations and averaging also over all directions provides the surface density in the form, In this way, we can only calculate σ ( z ) for integer values of z . For fractional z that are predicted from our evaluation of degenerate configurations in the next section, we use a linear interpolation to obtain . Equations (4) and (8) lead to a self-consistent equation for the average Voronoi volume in the form: . Analytic expressions for V * and S * can be derived in the spherical limit in closed form, where also the self-consistency equation can be solved exactly [20] . For non-spherical shapes we resort to a numerical integration to obtain V * and S *. Equation (4) can then be solved numerically, which yields , and subsequently the equation of state for the volume fraction versus coordination number, , in numerical form (denoting explicitly the dependence on α ). Variation of the coordination number with aspect ratio In this purely geometric theory of the average Voronoi volume, the packing fraction is given as ( z , α ), with z and α free parameters, in principle. In practice, z is fixed by the symmetry properties of the object shape, z ( α ), and the physical condition of mechanical stability, requiring force and torque balance on every particle. Under the assumption of minimal correlations, these conditions typically motivate the isostatic conjecture based on Maxwell's counting argument [31] : z =2 d f , with d f the number of degrees of freedom, giving z =6 for fully symmetric objects (spheres), z =10 for rotationally symmetric shapes like spherocylinders, dimers and ellipsoids of revolution [6] , and z =12 for shapes with three different axis like aspherical ellipsoids and tetrahedra [13] . While the isostatic conjecture is well-satisfied for spheres, packings of non-spherical objects are in general hypoconstrained with z< 2 d f , where z ( α ) increases smoothly from the spherical value for α >1 (ref. 6 ). The fact that these packings are still in a mechanically stable state can be understood in terms of the occurrence of stable degenerate configurations ( Fig. 5 ), which reduce the effective number of degrees of freedom [32] . However, the observed variation z ( α ) could not be explained quantitatively so far. Here we deduce the relation z ( α ) by evaluating the probability of finding these degenerate configurations to provide a prediction of ( α ) in close form. 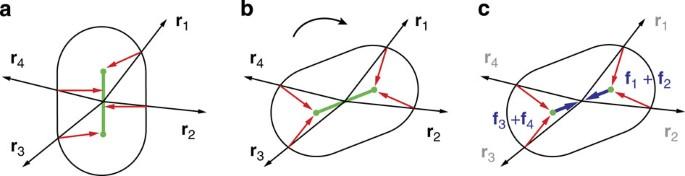Figure 5: Quantitative method to calculatez(α). (a) A 2D sketch of a spherocylinder with a random configuration of contact directionsrj. The associated forces are along directionsnormal to the surface (indicated in red) and torques are along. From these directions, one can determine if mechanical equilibrium has some redundancy, that is, if force and torque balance equations are not linearly independent. The configuration shown has no redundancy: The equivalent situation in three dimensions would show force and torque balance equations as five different constraints (the most general case for a 3D particle would be six constraints, but the torque along the axis of a spherocylinder is always vanishing, due to its rotational symmetry). (b) Here the spherocylinder is rotated. With the same contact directionsrjas ina, the contact force directionsare now modified. We explore the space of possible orientations for the spherocylinder, and try to find configurations which maximize redundancy in the mechanical equilibrium conditions. (c) As an example, this orientation exhibits some redundancy: All the contacts are on the spherical caps of the spherocylinder. Therefore,f1+f2andf3+f4are aligned with the spherocylinder axis and the condition of force balance automatically implies torque balance. If this is the orientation of the spherocylinder for which redundancy is maximal, we associate the number of linearly independent equations (that is, the effective number of degrees of freedom) from the mechanical equilibrium condition with the set of contact directions {rj} and perform an average over the possible sets of {rj}. This yields the averaged effective number of degrees of freedomfor a spherocylinder having an aspect ratioαand the coordination number follows as. Note that for non-convex shapes like dimers, the resultingzis the number of contacting neighbours, not the number of contacts, which can exceed the former. Figure 5: Quantitative method to calculate z ( α ). ( a ) A 2D sketch of a spherocylinder with a random configuration of contact directions r j . The associated forces are along directions normal to the surface (indicated in red) and torques are along . From these directions, one can determine if mechanical equilibrium has some redundancy, that is, if force and torque balance equations are not linearly independent. The configuration shown has no redundancy: The equivalent situation in three dimensions would show force and torque balance equations as five different constraints (the most general case for a 3D particle would be six constraints, but the torque along the axis of a spherocylinder is always vanishing, due to its rotational symmetry). ( b ) Here the spherocylinder is rotated. With the same contact directions r j as in a , the contact force directions are now modified. We explore the space of possible orientations for the spherocylinder, and try to find configurations which maximize redundancy in the mechanical equilibrium conditions. ( c ) As an example, this orientation exhibits some redundancy: All the contacts are on the spherical caps of the spherocylinder. Therefore, f 1 + f 2 and f 3 + f 4 are aligned with the spherocylinder axis and the condition of force balance automatically implies torque balance. If this is the orientation of the spherocylinder for which redundancy is maximal, we associate the number of linearly independent equations (that is, the effective number of degrees of freedom) from the mechanical equilibrium condition with the set of contact directions { r j } and perform an average over the possible sets of { r j }. This yields the averaged effective number of degrees of freedom for a spherocylinder having an aspect ratio α and the coordination number follows as . Note that for non-convex shapes like dimers, the resulting z is the number of contacting neighbours, not the number of contacts, which can exceed the former. Full size image In a degenerate configuration, force balance already implies torque balance, as the net forces are aligned with the inner axis of the particle ( Fig. 5 ). This implies that there is redundancy in the set of force and torque balance equations for mechanical equilibrium as force and torque balance equations are not linearly independent. Our evaluation of these degenerate configurations is based on the assumption that a particle is always found in an orientation such that the redundancy in the mechanical equilibrium conditions is maximal. This condition allows us to associate the number of linearly independent equations involved in mechanical equilibrium with the set of contact directions. Averaging over the possible sets of contact directions then yields the average effective number of degrees of freedom , from which the coordination number follows as (Methods). The results for z ( α ) are shown in Fig. 6a for prolate ellipsoids of revolution, spherocylinders, dimers and lens-shaped particles. We are able to recover the observed continuous transition as a function of α from the isostatic coordination number for spheres, z =6 at α =1, to the isostatic value z =10, for aspect ratios above ≈1.5. The trend compares well to known data for ellipsoids [6] and spherocylinders [10] , [17] . In particular, our approach explains the decrease of z for higher aspect ratios observed in simulations of spherocylinders [10] , [17] : For large α , the most probable case is to have contacts only on the cylindrical part of the particle, so that all normal forces are coplanar reducing the effective number of degrees of freedom by one. Consequently, z →8 as α →∞, as we obtain in Fig. 6a . This decrease is specific to spherocylinders, and not observed for dimers or ellipsoids, since the normal forces are not coplanar. 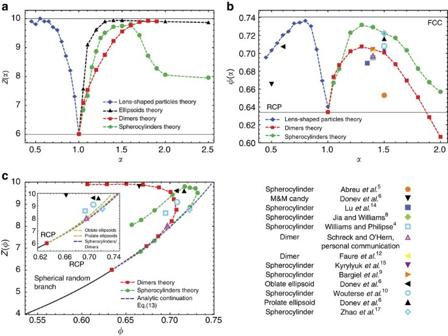Figure 6: Theoretical predictions for packings of particles with various shapes. (a) The functionz(α) determined by evaluating the probability of degenerate configurations. Both spherocylinders and dimers increase up to just below the isostatic valuez=10. For dimers,z(α) is the number of contacting neighbours, not the number of contacts, as a single contacting particle can have more than one contacting point. For spherocylinders,zreduces to 8 for largeα, as the forces acting on the cylindrical part are coplanar and reduce the effective degree of freedom. We also include the results from our method for prolate ellipsoids of revolution and lens-shaped particles. (b) The predicted packing fraction(α) of spherocylinders, dimers and lens-shaped particles compared with simulation results of maximal densities from the literature. We predict the maximal packing fraction of spherocylindersmax=0.731 atα=1.3 and of dimersmax=0.707 atα=1.3, demonstrating that spherocylinders pack better than dimers. For the lens-shaped particles we obtainmax=0.736 atα=0.8. (c) By plottingzvswe obtain a phase diagram for smooth shapes. We observe that the spherical random branchsph, which ends at the RCP point at (0.634,6) (ref.20), in fact continues smoothly upon deformation into dimers and spherocylinders as predicted by our theory. The spherocylinder continuation provides a boundary for all known packing states of rotationally symmetric shapes. Inset: The continuations from RCP. For a given value ofz, the densest packing is achieved by spherocylinders, followed by dimers, prolate ellipsoids and oblate ellipsoids. Note that the continuations for spherocylinders and dimers are almost identical. Figure 6: Theoretical predictions for packings of particles with various shapes. ( a ) The function z ( α ) determined by evaluating the probability of degenerate configurations. Both spherocylinders and dimers increase up to just below the isostatic value z =10. For dimers, z ( α ) is the number of contacting neighbours, not the number of contacts, as a single contacting particle can have more than one contacting point. For spherocylinders, z reduces to 8 for large α , as the forces acting on the cylindrical part are coplanar and reduce the effective degree of freedom. We also include the results from our method for prolate ellipsoids of revolution and lens-shaped particles. ( b ) The predicted packing fraction ( α ) of spherocylinders, dimers and lens-shaped particles compared with simulation results of maximal densities from the literature. We predict the maximal packing fraction of spherocylinders max =0.731 at α =1.3 and of dimers max =0.707 at α =1.3, demonstrating that spherocylinders pack better than dimers. For the lens-shaped particles we obtain max =0.736 at α =0.8. ( c ) By plotting z vs we obtain a phase diagram for smooth shapes. We observe that the spherical random branch sph , which ends at the RCP point at (0.634,6) (ref. 20 ), in fact continues smoothly upon deformation into dimers and spherocylinders as predicted by our theory. The spherocylinder continuation provides a boundary for all known packing states of rotationally symmetric shapes. Inset: The continuations from RCP. For a given value of z , the densest packing is achieved by spherocylinders, followed by dimers, prolate ellipsoids and oblate ellipsoids. Note that the continuations for spherocylinders and dimers are almost identical. Full size image Phase diagram of non-spherical particles Our calculation leads to a close theoretical prediction for the packing density ( α )= ( z ( α ), α ) which does not contain any adjustable parameters. Figure 6b shows the prediction for dimers, spherocylinders and lens-shaped particles. For spherocylinders, results in the literature on ( α ) vary greatly ( Table 1 ), but all show a peak at around α ≈1.3–1.5, which is captured by our formalism. We predict the maximum density of spherocylinders at α =1.3 with a density max =0.731 and that of dimers at α =1.3 with max =0.707. We have also calculated the packing fraction of the lens-shaped particles of Fig. 3c , which yields max =0.736 for α =0.8. This shape represents the densest random packing of an axisymmetric shape known so far. We further investigate packings of non-spherical objects in the z – representation. This change in perspective allows us to characterize packings of differently shaped objects in a phase diagram. By plotting z ( α ) against ( α ) parametrically as a function of α , we obtain a phase diagram for jammed anisotropic particles in the z – plane ( Fig. 6c ). In the same diagram, we also plot the equation of state obtained with the present theory in the case of spheres in [20] : , which is valid between the two isostatic limits of frictionless spheres z =6 and infinite frictional spheres at z =4. Surprisingly, we find that both dimer and spherocylinder packings follow an analytical continuation of these spherical packings. This result highlights that the spherical random branch can be continued smoothly beyond the RCP in the z – plane. The analytical continuation of RCP is derived by solving the self-consistent equation (4) close to the spherical limit ( Supplementary Methods ): here denotes the spherical free-volume at RCP defined as evaluated at z =6 as calculated in [20] , is the spherical isostatic value, and the functions g 1,2 can be expressed in terms of exponential integrals. The dependence of equation (13) on the object shape is entirely contained in the geometrical parameters M b , M v , and M z : M b and M v quantify the first-order deviation from the sphere at α =1 of the object's hard-core boundary and its volume, respectively, while M z measures the first-order change in the coordination number upon deformation of the sphere. The resulting continuations z ( ) obtained by inverting equation (13) for different object shapes are plotted in the inset of Fig. 6c . For the smooth shapes considered, we find generally that denser packing states are reached for higher coordination numbers. For a given value of z , spherocylinders achieve the densest packing, followed by dimers, prolate ellipsoids and oblate ellipsoids, as seen in the inset of Fig. 6c . We observe that the densest packing states for dimers and spherocylinders found in simulations lie almost exactly on the continuation, while the one of the ellipsoids deviate considerably. Comparison with empirical data Table 1 indicates that there is a finite range of densities for random jammed packings according to the particular experimental or numerical protocol used (denoted as a J-line in the case of jammed spheres [19] , [33] ). On the other hand, our mean-field theory predicts a single density value and Fig. 6 indicates that our predictions are an upper bound of the empirical results. We interpret these results in terms of current views of the jamming problem developed in the limiting case of spheres, where the question of protocol-dependency of packings has been systematically investigated. Random close packings can be considered as infinite-pressure limits of metastable glass states, which was shown theoretically in refs 19 , 34 , 35 , 36 and confirmed in computer simulations in ref. 37 . Indeed, there exist a range of packing fractions named as [ th , GCP ] following the notation of mean-field Replica Theory (RT) [19] . Here GCP stands for the density of the ideal glass close packing and is the maximum density of disordered packings, while t h is the infinite-pressure limit of the least dense metastable states. In RT, the states [ th , GCP ] are all isostatic. From the point of view of simulations, the well-known Lubachevsky–Stillinger (LS) protocol [33] provides this range of packings for different compression rates. The densities [ t h , GCP ] are achieved by the corresponding compression rates (from large to small) [ γ th , γ GCP →0]. Compression rates larger than γ th all end to th . The threshold value γ th corresponds to the relaxation time 1/ γ th of the least dense metastable glass states. The denser states at GCP are unreachable by experimental or numerically generated packings, as it requires to equilibrate the system in the ideal glass phase, a region where the relaxation time is infinite. In general, large compression rates lead to lower packing fractions. This picture was investigated for sphere packings in [33] , [38] and it is particularly valid for high-dimensional systems where crystallization is avoided [19] . Random close packings are also known to display sharp structural changes [39] , [40] , [41] , [42] , [43] signalling the onset of crystallization at a freezing point c (ref. 18 ). All the (maximally random) jammed states along the segment [ th , GCP ] can be made denser at the cost of introducing some partial crystalline order. Support for a order/disorder transition at c is also obtained from the increase of polytetrahedral substructures up to RCP and its consequent decrease upon crystallization [44] . In terms of protocol preparation like the LS algorithm, there exists a typical time scale t c corresponding to crystallization. Crystallization appears in LS [18] , [19] , [41] if the compression rate is smaller than γ c =1/ t c , around the freezing packing fraction [45] . A possible path to avoid crystallization and obtain RCP in the segment [ th , GCP ] is to equilibrate with γ > γ c to pass the freezing point, and eventually setting the compression rate in the range [ γ th , γ GCP →0] to achieve higher volume fraction. As the present statistical mechanics framework is based on the Edwards ensemble approach [27] , our prediction of the packing density Edw corresponds to the ensemble average over the configuration space of random states at a fixed coordination number. As the volume has the role of the Hamiltonian, the energy minimization in equilibrium statistical mechanics is replaced in our formalism by a volume minimization: The highest volume fraction for a given disordered system is achieved in the limit of zero compactivity. Therefore, the present framework provides a mean-field estimation of such a maximal volume fraction (minimum volume) of random packings with no crystallization. As we perform an ensemble average over all packings at a fix coordination number, the obtained volume fraction Edw corresponds to the one with the largest entropy (called largest complexity in RT) along [ th , GCP ]. This point needs not to be th , and in general it is a larger volume fraction. Thus, . The above discussion can be translated to the present case of non-spherical particles. In this case, unfortunately, there is no detailed study of the protocol-dependent packing density as done by [19] , [33] , [38] for spheres. However, the survey of the available simulated data obtained by different groups ( Table 1 and Fig. 6b ) can be interpreted analogously as for spheres. In the case of spherocylinders, packings have been obtained in the range [0.653, 0.722] (these minimum and maximum values have been obtained in ref. 5 and in ref. 17 , respectively, see Table 1 ). Our predicted density is 0.731, representing an upper bound to the simulated results. In the case of dimers, there are two simulations giving a density of 0.697 (C. F. Schreck and C. S. O'Hern (2011) personal communication) and 0.703 (ref. 12 ), which are both smaller than and very close to our prediction 0.707. Thus, our prediction is interpreted as the upper limit in the range of packings observed with numerical algorithms. Under this scenario, which is consistent with analogous three-dimensional (3D) spherical results, packings may exist in the region [ th , Edw ], and our theory is a mean-field estimation of Edw . This region is very small for spheres but the above evidence indicates that non-spherical particles may pack randomly in a broader range of volumes. The present framework estimates the upper bound for such a range. We would like to stress that our analytic continuation is non-rigorous and appears as the solution of our mean-field theory for first-order deviations in α from the sphere using suitable approximations. The shapes of dimers, spherocylinders, ellipsoids are then all shown to increase the density of the random packing to first-order. In the case of regular (crystal) packings, recent mathematically rigorous work has shown in fact that for axisymmetric particles any small deformation from the sphere will lead to an increase in the optimal packing fraction of the crystal [46] . This appears only in 3D and is related to Ulam's conjecture stating that the sphere is the worst case scenario for ordered packings in 3D (ref. 47 ). A full mathematical proof of this conjecture is still outstanding, but so far all computer simulations verify the conjecture. In particular, recent advances in simulation techniques allow to generate crystal packings of a large variety of convex and non-convex objects in an efficient manner [48] , [49] . The extensive study of de Graaf et al . [48] has extended the verification of Ulam's conjecture to the first eight regular prisms and antiprisms, the 92 Johnson solids, and the 13 Catalan solids. The verification for regular n -prisms and n -antiprisms can be extended to arbitrary n using this method, providing an exhaustive empirical verification of the conjecture for these regular shapes. We remark that a random analogue of Ulam's packing conjecture has been proposed and verified for the Platonic solids (apart from the cube) in simulations [16] . The results presented here support the random version of Ulam's conjecture and might help in investigating this conjecture further from a theoretical point of view. We believe that our decomposition of various shapes into intersections and overlaps of spheres will be a useful starting point for a systematic investigation of this issue. Our approach can be systematically continued beyond the axisymmetric shapes considered here. For instance, in Fig. 2e–h , we have 2,3,6,n anti-points to describe ellipsoids and polyhedra of increasingly varying complexity. The challenge would be to implement our algorithm to calculate the resulting Voronoi excluded volumes that appear in our mean-field theory. For this, one might also consider a fully numerical evaluation using, for example, graphics hardware [25] . Quantitative method to calculate z ( α ) Mathematically, we can write the local mechanical equilibrium on a generic non-spherical frictionless particle having k contacts defined by their location r j , normal and force , as: where is a matrix. A local degenerate configuration has a matrix such that . We base our evaluation on two assumptions: (i) Contact directions around a particle in the packing are uncorrelated, and (ii) Given one set of contact directions, a particle i is found in an orientation such that the redundancy in the mechanical equilibrium conditions is maximal, that is, is a minimum. Note that depends on , as only the absolute direction of contact points are chosen, and thus rotating particle i affects the direction and normal of these contacts with respect to particle i . This situation is described in Fig. 5c , which includes a two-dimensional (2D) sketch of a 3D degenerate configuration that we observe often in our procedure. In this case, the rank is reduced by one unit, and the probability of occurrence of such a situation is large at small aspect ratio, as it just requires that there is no contact on the cylindrical part of the inner particle. Within our assumptions, we explore the space of possible contact directions for one particle, given a local contact number k , and aspect ratio α . We then extract the average effective number of degrees of freedom , which is the average over the contact directions of the minimal value of : , where denotes the average over contact directions. This average is limited to a subset J of all possible { r 1 … r k } such that mechanical equilibrium (equation 14) is possible with positive forces, as expected for a packing of hard particles. This corresponds geometrically to sets { r 1 ,…, r k } which do not leave a hemisphere free on the unit sphere. Finally, the normalization is the volume of J . For a packing with a coordination number distribution Q z ( k ), with average z , the effective d f is: , and the average z follows as . In our evaluation, we use a Gaussian distribution for Q z ( k ), with variance 1.2 and average z , consistent with simulations [50] . Overall, z ( α ) is thus the solution of the following self-consistent relation: The way we look for the orientation on the unit sphere showing the lowest rank is simply by sampling it randomly with a uniform distribution (10 6 samples). The computation of the rank is done via a standard Singular Value Decomposition of , which is here numerically accurate for α ≥1.05. Test of the approximations of the theory We perform a comprehensive test of the different approximations of the theory using computer simulations of spherocylinder packings ( Supplementary Note 1 ). From the generated configurations at the jamming point we obtain the CDF P ( c , z ), where z is also an observable of the simulation determined by the jamming condition. P ( c , z ) contains the probability that the boundary of the Voronoi volume in the direction is found at a value larger than c and is determined as follows. We select an orientation relative to the orientation of a chosen reference particle i . A large number of particles in the packing contribute a VB along with particle i . We determine all these different VBs denoted by . The boundary of the Voronoi volume in the direction is the minimum c m of all positive VBs: where r j and are the relative position and orientation of particle j with respect to the reference particle i . Determining this minimal VB for all particles i in the packing yields a list of c m values for a given (which is always relative to the orientation ). The CDF P ( c , z ) simply follows by counting the number of values larger than a specified c . Owing to the rotational symmetry of the spherocylinders, the orientational dependence of P ( c , z ) is reduced to P ( c , θ c ; z ), where θ c is the polar angle of the orientation in spherical coordinates. Moreover, due to inversion symmetry it is sufficient to select only . Therefore, we choose three θ c values to cover this range: θ c =0.22, 0.8, 1.51. We also use the rotational symmetry to improve the sampling of P ( c , z ): We fix θ c to one of the three values, but select a number of azimuthal angles at random. As the packing is statistically isotropic for all azimuthal angles, the resulting c m value for these directions can all be included in the same ensemble. We consider three different aspect ratios α =1.1, 1.5, 2.0 of the spherocylinders to capture a range of different shapes. The results are plotted in Fig. 7 . 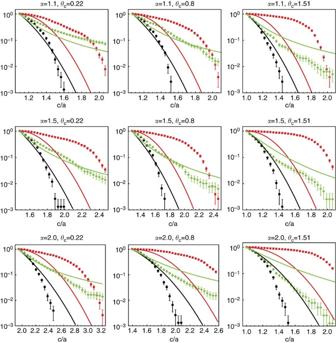Figure 7: Comparison of the CDF with simulation data. We plot the theoretical predictions (solid lines) forP(c,z) (black),PB(c) (red) andPC(c,z) (green) with the corresponding CDFs sampled from simulated configurations (symbols) of spherocylinders. For each aspect ratioα=1.1, 1.5, 2.0, we plot results for three values of the polar angleθc[0,π/2]. We generally observe that the three CDFs agree quite well in the regime of smallcvalues, which provides the dominant contribution to the average Voronoi volume. The same plots are shown on a linear scale in theSupplementary Fig. S1. The error bars denote the root mean square error of the finite-size sampling. Figure 7: Comparison of the CDF with simulation data. We plot the theoretical predictions (solid lines) for P ( c , z ) (black), P B ( c ) (red) and P C ( c , z ) (green) with the corresponding CDFs sampled from simulated configurations (symbols) of spherocylinders. For each aspect ratio α =1.1, 1.5, 2.0, we plot results for three values of the polar angle θ c [0, π /2]. We generally observe that the three CDFs agree quite well in the regime of small c values, which provides the dominant contribution to the average Voronoi volume . The same plots are shown on a linear scale in the Supplementary Fig. S1 . The error bars denote the root mean square error of the finite-size sampling. Full size image We test the two main approximations considered in the theory: (a) The derivation of P ( c , z ) using a liquid like theory of correlations as done in Song et al . [20] Jin et al . [29] leading to the exponential form of equation (8). (b) The factorization of this CDF into contact and bulk contributions as in equation (11). This approximation neglects the correlations between the contacting particles and the bulk. In Fig. 7 , we test these approximations by comparing theory and simulations for three different CDFs: P ( c , z ), P B ( c ) and P C ( c , z ), equations (8)–(10),. In order to determine the P B ( c ) from the simulation data we need to take the contact radius between particle i and any particle j into account. The minimal VB, c m , is determined from the contributed VBs of particles in the bulk only, that is, particles with . Likewise, P C ( c ) is determined from the simulation data by only considering VBs of contacting particles with . Following this procedure, we have tested these approximations with the computer generated packings. We find ( Fig. 7 ): (i) The contact term P C is well approximated by the theory for the full range of c ; (ii) For small values of c the bulk distribution P B is well approximated by the theory, and deviations are observed for larger c ; (iii) The full CDF P ( c ) agrees well between the computer simulations and the theory, especially for small c . The small values of c provide the dominant contribution in the self-consistent equation to calculate the average Voronoi volume equation (4), and therefore to the main quantity of interest, the volume fraction of the packing. This can be seen by rewriting equation (4) as as the CDF is trivially unity for c values smaller than the hard-core boundary . The main contribution to the integral then comes from c values close to due to the decay of the CDF. Systematic deviations in our approximations arise in the bulk distribution P B for larger values of c , but, interestingly, the slope of the decay still agrees with our theory. Overall, the comparison highlights the mean-field character of our theory: Correlations are captured well up to about the first coordination shell of particles, after which theory and simulations diverge, especially for the bulk term. The agreement is acceptable for the nearest neighbour-shell, but is incorrect for the second neighbours. Beyond this shell, bulk particles are affected in a finite range by correlations that we do not address, as we assume a uniform distribution of the density of these particles; this is a typical assumption in a mean-field theory. The additional unaccounted correlations lead to a slightly higher probability to observe the VB at intermediate c values in the simulation, compared with our theory. However, these deviations from simulations are small. For instance, Fig. 7 indicates that for a typical value α =1.5 and polar angle θ S =0.22, the numerically measured CDF P ( c , z ) at a relative large value c / a =2 is of the order of 10 −3 , while the theory predicts this probability at a slightly larger value of c / a =2.07. This small discrepancy is not relevant, as such a value of the probability is negligibly small in the calculation of the volume fraction in equation (4). Thus, because of this small probability to find the VB with values larger than c / a =2, the deviations expected from our approximations are small. These results indicate that, overall, the theory captures the distribution of VBs in the region of small c , which is the relevant region in the calculation of the volume fraction. The neglected higher-order correlations in the upper coordination shells can only decrease the volume fraction in the calculation leading to smaller packing densities. Following this analysis, we interpret our predicted packing fractions as upper bounds for the empirically found ones, which is indeed observed in Fig. 6b . How to cite this article: Baule, A. et al . Mean-field theory of random close packings of axisymmetric particles. Nat. Commun. 4:2194 doi: 10.1038/ncomms3194 (2013).